Genome-wide association study identifies variation at 6q25.1 associated with survival in multiple myeloma Survival following a diagnosis of multiple myeloma (MM) varies between patients and some of these differences may be a consequence of inherited genetic variation. In this study, to identify genetic markers associated with MM overall survival (MM-OS), we conduct a meta-analysis of four patient series of European ancestry, totalling 3,256 patients with 1,200 MM-associated deaths. Each series is genotyped for ∼ 600,000 single nucleotide polymorphisms across the genome; genotypes for six million common variants are imputed using 1000 Genomes Project and UK10K as the reference. The association between genotype and OS is assessed by Cox proportional hazards model adjusting for age, sex, International staging system and treatment. We identify a locus at 6q25.1 marked by rs12374648 associated with MM-OS (hazard ratio=1.34, 95% confidence interval=1.22–1.48, P =4.69 × 10 –9 ). Our findings have potential clinical implications since they demonstrate that inherited genotypes can provide prognostic information in addition to conventional tumor acquired prognostic factors. Multiple myeloma (MM) is a malignancy characterized by the infiltration of clonal plasma cells in the bone marrow [1] , [2] . There is considerable heterogeneity in the survival outcomes among MM patients and a variety of clinical features and tumour biomarkers have been shown to be predictive of prognosis [3] , [4] , [5] , [6] , [7] , [8] . As a potential prognostic factor, the concept of germline variation imparting inter-individual variability in tumour development and progression is receiving increasing attention [9] , [10] , [11] , [12] . This observation is exemplified by breast cancer where a more accurate assessment of prognosis can be made by taking into account genetic information to improve therapeutic decision making, opening up the possibility of patient-tailored drug selection decisions [13] . In addition, detecting genes with prognostic relevance has the potential to aid the identification of pathways that could be targeted for novel therapeutic interventions. Here to identify germline variation influencing patient outcome following a diagnosis of MM we have pooled genotype data from four independent genome-wide association studies (GWAS) of MM [14] , [15] , [16] , [17] and linked these to survival time data. Our findings are consistent with the hypothesis that an individual’s prognosis following treatment for MM is influenced by germline variation. Specifically, we identified a locus at 6q25.1 (rs12374648) associated with MM-OS that was statistically significant. Moreover, the association at 6q25.1 was consistently seen in each of the four patient cohorts and was not confined to a specific molecular subtype of MM. Genome-wide association study After applying quality control measures, genotype data were available on 3,256 cases from the GWAS series, Supplementary Figs 1 and 2 . The inflation factor four λ for each of the studies ranged from 0.99 to 1.03 and for the overall analysis was 1.02 ( Supplementary Figs 3 and 4 ). We identified eight single nucleotide polymorphisms (SNPs) associated with MM-OS at P values ≤5.0 × 10 −8 ; proportional hazards model. All eight SNPs were located on chromosome 6q25.1 and were in linkage disequilibrium ( r 2 =0.58–1.0), Figs 1 and 2 . 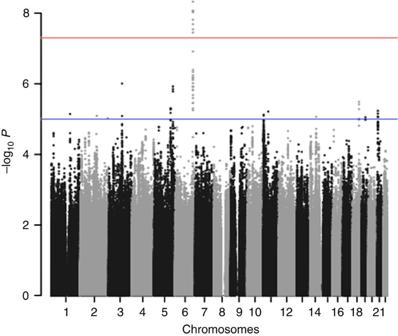Figure 1: Association plot for combined analyses for MM-OS. TheP-values of the association between each SNP and myeloma survival were obtained by Cox regression analyses with adjustment and then combined. Theyaxis shows the −log10P-values of each SNP analysed, and thexaxis shows their respective chromosome position. The red horizontal line corresponds toP=5.0 × 10−8. All statistical tests were two-sided. The strongest association was provided by rs12748648 ( P =4.89 × 10 −9 , hazard ratio (HR)=1.34, 95% confidence interval (CI)=1.22–1.48, risk allele frequency=0.19); Table 1 , Fig. 2 and Supplementary Fig. 5 . The association was consistent across the four series and there was very little between-study heterogeneity ( P =0.34, I 2 =11%; test of heterogeneity). Homozygosity for rs12748648 GG was associated with median survival time of 26.7 (UK-My9), 42.8 (GER-German-speaking Myeloma Multicenter Study Group (GMMG)) and 80 (US-University of Arkansas for Medical Sciences (UAMS)) months as compared with 60, 92.2 and 137 months, respectively, for patients homozygous for AA genotype ( Fig. 3 ). To address the possibility that the impact of rs12748648 on MM-OS is a consequence of its association with known cytogenetic risk factors we performed a multivariate analysis on the 1,165 patients of the UK-My9 cohort including rs12748648, high-risk IgH translocations, gain(1q21) and del(17p). This showed that 6p25.1 (rs12374648) independently impacted MM-OS ( Supplementary Table 1 ). Patients with complete remission after autologous cell transplant (ASCT) tend to have a better survival. We examined whether the 6q25.1 association for OS was confined to patients with or without complete remission and we found the association was apparent in both patient groups ( P =0.84; test of heterogeneity). Figure 1: Association plot for combined analyses for MM-OS. The P -values of the association between each SNP and myeloma survival were obtained by Cox regression analyses with adjustment and then combined. The y axis shows the −log 10 P -values of each SNP analysed, and the x axis shows their respective chromosome position. The red horizontal line corresponds to P =5.0 × 10 −8 . All statistical tests were two-sided. 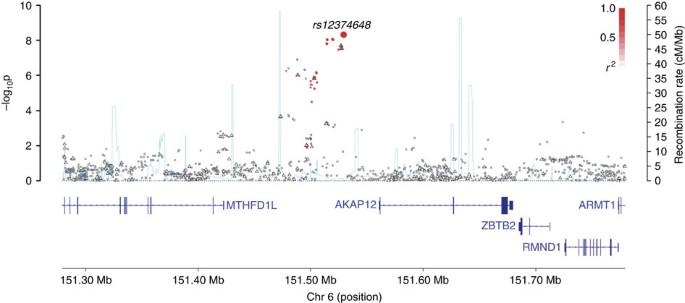Figure 2: Regional plot of association results and recombination rates for the rs12374648 (6q25.1) MM-OS risk locus. Plots show association results of both genotyped (triangles) and imputed (circles) SNPs in the GWAS samples and recombination rates. −log10P-values (yaxes) of the SNPs are shown according to their chromosomal positions (xaxes). The top genotyped SNP in each combined analysis is shown as a large diamond and is labelled by its rsID. The colour intensity of each symbol reflects the extent of LD with the top genotyped SNP, white (r2=0) through to dark red (r2=1.0). Genetic recombination rates, estimated using HapMap samples from Utah residents of western and northern European ancestry (CEU), are shown with a light blue line. Physical positions are based on NCBI build 37 of the human genome. Also shown are the relative positions of genes and transcripts mapping to the region of association. Genes have been redrawn to show their relative positions; therefore, maps are not to physical scale. Below each plot is a diagram of the exons and introns of the genes of interest. Full size image Figure 2: Regional plot of association results and recombination rates for the rs12374648 (6q25.1) MM-OS risk locus. Plots show association results of both genotyped (triangles) and imputed (circles) SNPs in the GWAS samples and recombination rates. −log 10 P -values ( y axes) of the SNPs are shown according to their chromosomal positions ( x axes). The top genotyped SNP in each combined analysis is shown as a large diamond and is labelled by its rsID. The colour intensity of each symbol reflects the extent of LD with the top genotyped SNP, white ( r 2 =0) through to dark red ( r 2 =1.0). Genetic recombination rates, estimated using HapMap samples from Utah residents of western and northern European ancestry (CEU), are shown with a light blue line. Physical positions are based on NCBI build 37 of the human genome. Also shown are the relative positions of genes and transcripts mapping to the region of association. Genes have been redrawn to show their relative positions; therefore, maps are not to physical scale. Below each plot is a diagram of the exons and introns of the genes of interest. Full size image Table 1 Summary result for the combined analysis of 6q25.1 (rs12374648) and MM-OS. 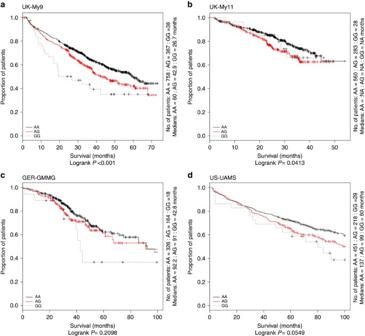Figure 3: Kaplan–Meier curves for MM-OS at 6q25.1 (rs12374648). Survival curves for the AA homozygotes are shown as a solid line. The red line depicts the survival curve for the AG heterozygotes, and the dashed line depicts the survival curve for the rare homozygotes GG. Vertical ticks indicate censored data points. Full size table Figure 3: Kaplan–Meier curves for MM-OS at 6q25.1 (rs12374648). Survival curves for the AA homozygotes are shown as a solid line. The red line depicts the survival curve for the AG heterozygotes, and the dashed line depicts the survival curve for the rare homozygotes GG. Vertical ticks indicate censored data points. Full size image Overall survival risk allele for myeloma at 6p25.1 rs12748648 maps within a 49.2-Kb ( r 2 >0.2) region of linkage disequilibrium intergenic to MTHFD1L and AKAP12 genes ( Fig. 2 ). The genomic region contains multiple enhancer marks and the SNP localizes to a predicted enhancer element that is bound by TCF4 (TCF7L2), Supplementary Fig. 5 . Analysis of eQTL data did not demonstrate a relationship between rs12748648 genotype and expression of MTHFD1L , AKAP12 or distantly flanking genes ( Supplementary Figs 6 and 7 ). Examining encyclopedia of DNA elements (ENCODE) CHIP-seq data in the lymphoblast cell line GM12878 of the 6p25.1 showed that rs12748648 maps to region enriched for H3K27me3, a polycomb repressive mark. As DNA methylation can have a role in access of such polycomb repression [18] , we undertook a meQTL analysis of the region around rs12748648. We found an association between rs12748648 risk genotype and reduced methylation of both MTHFD1L and AKAP12 genes ( P =0.0077 and 0.0097, respectively, log-linear regression; Supplementary Fig. 8 ). In addition to the 6q25.1 (rs12748648) association for MM-OS we identified suggestive associations (that is P <10 −5 ; proportional hazards model) at 1q23.3 (rs1934908), 19q13.11 (rs1974807), 5q31.3 (rs2906053), 3q13 (rs4682170), 18q21 (rs57942319) and 2q22 (rs61070260; Supplementary Table 2 and Supplementary Figs 9–20 ). All of the SNPs defining these associations mapped to genomic regions with regulatory marks ( Supplementary Table 3 ), with rs1934908 impacting FCLRA expression in plasma cells ( Supplementary Fig. 21 ). All of the SNP associations noted above for MM-OS showed a consistent effect on progression-free survival, Supplementary Table 4 . It is possible that some of the inherited genetic variants that impact on the risk of developing MM [14] , [16] , [17] , [19] , may also impact on MM-OS. To address this possibility we examined the relationship between previously published risk SNPs and MM-OS. None of the nine validated risk SNPs for MM were associated with MM-OS, that is, P >0.05, proportional hazards model; Supplementary Table 5 . Our findings suggest a hypothesis that an individual’s prognosis following treatment for MM is influenced by germline variation. In our analysis we adjusted for the influence of treatment on survival within studies, and report associations consistent across the four studies, thus our findings are likely to relate to underlying biology impacting the survival of the myeloma clone. The treatment used in all of the studies included ASCT, the GMMG studies used a tandem transplant, younger patients in the Medical Research Council (MRC) study received a single ASCT in both the Myeloma IX (UK-My9) and Myeloma IX (UK-My11) cases. The UAMS (US-UAMS) cases received predominantly tandem transplants together with combination induction and consolidation therapy. Prognostic factors generated from these studies are generally applicable to patients treated with ASCT and the use of novel agents including lenalidomide and bortezomib used as both induction and maintenance. The 6q25.1 locus that associates with MM-OS spans a region of LD intergenic to MTHFD1L and AKAP12 genes. While variation at 6q25.1 has previously been linked to coronary heart disease [20] , [21] (rs6922269) and late-onset Alzheimer disease [22] (rs11754661) the risk SNPs for these diseases are not correlated with rs12574648 (respective LD metrics– r 2 =0.002, D ′=0.08 and r 2 =0.046, D ′=0.65). MTHFD1L is involved in mitochondrial tetrahydrofolate (THF) synthesis [23] , [24] . One-carbon substituted forms of THF are important for the de novo synthesis of purines and thymidylate supporting cellular methylation by regenerating methionine from homocysteine. There have been no previous reports of associations of cancer risk or overall survival (OS) with variation at AKAP12 , but AKAP12 has been shown to be a tumour suppressor, acting through CyclinD1 (ref. 25 ). AKAP12 is regulated by methylation in a number of cancers [26] , [27] , [28] , [29] , [30] , [31] , [32] , [33] and is epigenetically repressed in MM, where its expression can be upregulated following treatment with DNA demethylation compounds such as trichostatin and/or 5-aza-2′-deoxycytidine [34] . Intriguingly, although rare, 6q is a site of recurrent deletion in lymphoid tumours, that includes homozygous deletions at 6q25.3 ( AR1D1B/WTAP ) [35] and mutations at 6q21 ( PRDM1/BLIMP1 ) [36] , [37] , [38] . It is however unlikely that any somatic mutations in this regions are responsible for the MM-OS signal. While the functional basis for the rs12374648 remains to be established the SNP maps to a binding site for the transcription factor TCF7L2, alias TCF4. Binding of TCF7L2 correlates with hypomethylation and contributes to formation of differentially methylated regions of the genome [39] ; TCF7L2 is commonly bound close to loci that are demethylated during differentiation [40] , [41] . Although speculative, we note that the rs12374648 risk genotype was associated with hypomethylation at the genomic region encompassing MTHFD1L and AKAP12 , suggesting a possible mechanistic basis for the 6q25.1 association. In addition to variation at 6q25.1, we identified suggestive associations at six other loci, a number of which annotate genes having strong a priori evidence for having a role in MM. Notably at 1q23.3, a region commonly amplified in MM, an association with rs1934908 genotype is also seen to be an eQTL for FRCLA , a gene with regulatory influence on IgG levels [42] . In contrast to these suggestive associations we did not find any evidence to support the recent claim that variation at 16p13 defined by the rare SNP rs72773978 influences the risk of MM-OS [43] , P combined =0.92, proportional hazards model; Supplementary Table 6 . GWASs have been successful in identifying variants influencing susceptibility for most cancers. Notably, nine common variants have thus far been shown to be associated with MM risk [14] , [15] , [16] , [17] , [19] . Paradoxically variants for cancer prognosis have been elusive and in this study we have only identified one variant for myeloma survival at genome-wide statistical significance. A major reason for the disparity is study power. Despite the size of our study, the power to detect association with MM-OS is at best only modest. All of the common susceptibility alleles for MM are associated with relative risks of ∼ 1.15 and such alleles can be identified through large case-control series, in contrast our survival analysis, based on 1,200 myeloma related deaths, had only 80% power to detect alleles with a HR greater ≥1.5 and minor allele frequency (MAF) >0.2. Our findings support the hypothesis that germline variation influences outcome following treatment of MM. These results provide insight into the molecular mechanisms of tumour progression implying that germline markers of prognosis have the potential to enhance risk stratification. However, it is clear that trials larger than ours are required to identify additional loci associated with OS. Genotyping samples from future clinical trials, is likely to be especially informative and to offer the prospect of establishing the relationship between inherited variants, molecular subtypes and specific therapies. Myeloma patient samples We pooled data from four independent MM case series [14] , [15] , [16] , [17] in populations of European ancestry with existing high-density SNP genotyping ( Supplementary Fig. 1 ): (i) UK-My11-GWAS comprising 877 MM cases from the UK MRC Myeloma IX trial. (ii) UK-My9-GWAS comprising 1,165 MM cases from the UK MRC Myeloma IX trial; (iii) German-GMMG-GWAS, comprising 511 MM patients recruited by the GMMG, coordinated by the University Clinic, Heidelberg; (iv) US-UAMS-GWAS comprising 703 newly diagnosed MM patients treated at the Myeloma Institute at UAMS. All of these trials have been reported previously but importantly all include a single or double autologous stem cell transplant as one component of the treatment [44] , [45] , [46] , [47] ( Table 2 ). All studies were approved by the relevant institutional review boards, and all participants provided written informed consent. Table 2 Clinical characteristics in the four patient cohorts. Full size table Genotyping and quality control Cases were genotyped using Illumina Human OmniExpress-12 v1.0 arrays according to the manufacturer’s protocols (Illumina, San Diego, USA). Standard quality control was performed on all scans, excluding individuals with low call rate (<90%) and extremely high or low heterozygosity ( P< 1.0 × 10 −4 , test of heterogeneity), as well as all individuals evaluated to be of non-European ancestry (using the HapMap version 2 CEU, JPT/CHB and YRI populations as a reference; Supplementary Fig. 2 ). A summary of the number of genotyped SNPs and the number of SNPs passing QC is detailed in Supplementary Fig. 1 . Imputation Genotypes for common variants across the genome were imputed using 1000 Genomes Project (phase 1 integrated release 3, March 2012) and UK10K as reference in conjunction with IMPUTE2 v2.1.1 (ref. 48 ) after pre-phasing with SHAPEIT software [49] . Poorly imputed SNPs defined by an information measure (Is)<0.90 were excluded from the analyses. All genomic locations are given in NCBI Build 37/UCSC hg19 coordinates. Statistical analysis The primary end point was MM-specific OS (MM-OS). Time-to-event was calculated from date of recruitment (left censoring) to avoid bias from the inclusion of prevalent cases. In the German series, the follow-up was started from transplantation, shortly after diagnosis. Follow-up was right censored on the date of death if death was other than MM, or the date last known alive if death did not occur. Kaplan–Meier survival curves according to genotype were generated and the homogeneity of the survival curves between genotypes was examined. Cox regression analysis was used to estimate genotype-specific HR and associated 95% CI. Where necessary we controlled for cryptic population substructure by including a variable number of principal components as covariates for each data set. For each SNP HRs were generated using common allele homozygotes as the reference group. P -values presented correspond to the significance of a test difference among all three of the genotype groups (common allele homozygote, heterozygote and rare allele homozygote). For SNPs where fewer than five minor allele homozygotes were observed, minor allele homozygote genotypes were combined with the heterozygotes. For the statistically significantly associated SNPs, we ran multivariable Cox models adjusting for ISS, age and treatment where appropriate. We confined our analysis to SNPs with MAF >5% because of extreme value of the test statistics. Overall statistical significance tests for each SNP were performed by combining the results for each data set using a fixed-effects meta-analysis. All statistical tests were two-sided. Inflation of the test statistics, λ , was estimated by dividing the 45th percentile of the test statistic by 0.357—the 45th percentile for a χ 2 distribution on 1 degree of freedom. Heterogeneity between studies was quantified using the I 2 statistic. Associations were regarded as statistically significant at a P value ≤5.0 × 10 –8 (that is, genome-wide significance). Multivariable stepwise variable selection was performed using a standard backward-elimination approach, variables were retained at a level of significance P <0.05. All statistical analyses were performed using R (v3.1.3) software [50] , [51] . eQTL analysis Expression quantitative trait locus (eQTL) analyses were performed for all genes in the 1 MB region spanning the MM-OS associated SNPs using Affymetrix Human Genome U133+2.0 array data for plasma cells from 184 MRC Myeloma IX trial patients, 658 GMMG patients and 604 UAMS patients, analysis as previously described [52] . In addition, we surveyed the effect of genotype on expression in other tissues using the publicly accessible GTeX (ref. 53 ), Blood eQTL (ref. 54 ), MuTHER studies [55] , Framingham heart study [56] and SCAN (ref. 57 ) databases. meQTL analysis Methylation quantitative trait locus analyses of adjacent genes to SNPs of interest using probe-level DNA methylation data generated using Illumina 450 K methylation arrays on plasma cells from 365 MRC myeloma XI trial patients (UK-My11). Association between SNP genotype and normalized methylation levels was tested by linear regression. Translocation detection Conventional cytogenetic studies of MM cells were conducted using standard karyotyping methodologies, and standard criteria for the definition of a clone were applied. Fluorescence in situ hybridization and ploidy classification of UK samples was conducted using methodologies previously described [58] , [59] . Fluorescence in situ hybridization and ploidy classification of GMMG samples was performed as previously described. The XL IGH Break Apart probe (MetaSystems, Altlussheim Germany) was used to detect any IGH translocation in GMMG [60] . Bioinformatics To explore the epigenetic profile of association signals, we used chromatin state segmentation in lymphoblastoid cell lines (LCL) data generated by the ENCODE project. The states were inferred from ENCODE histone modification data (histone H4 Lys20 methylation (H4K20me1), H3 Lys9 acetylation (H3K9ac), H3K4me3, H3K4me2, H3K4me1, H3K36me3, H3K27me3, H3K27ac and CCCTC-binding factor (CTCF)) binarized using a multivariate hidden Markov model. We used HaploReg and RegulomeDB [61] , [62] to examine whether any of the SNPs or their proxies (that is, r 2 >0.8 in the 1000 Genomes EUR reference panel) annotating putative transcription factor binding or enhancer elements. We assessed sequence conservation using Genomic Evolutionary Rate Profiling scores [63] . How to cite this article: Johnson, D. C. et al . Genome-wide association study identifies variation at 6q25.1 associated with survival in multiple myeloma. Nat. Commun. 7:10290 doi: 10.1038/ncomms10290 (2016).